One-way transparency of four-coloured spin-wave excitations in multiferroic materials The coupling between spins and electric dipoles governs magnetoelectric phenomena in multiferroics. The dynamical magnetoelectric effect, which is an inherent attribute of the spin excitations in multiferroics, drastically changes the optical properties of these compounds compared with conventional materials where light-matter interaction is expressed only by the dielectric permittivity or magnetic permeability. Here we show via polarized terahertz spectroscopy studies on multiferroic Ca 2 CoSi 2 O 7 , Sr 2 CoSi 2 O 7 and Ba 2 CoGe 2 O 7 that such magnetoeletric spin excitations exhibit quadrochroism, that is, they have different colours for all the four combinations of the two propagation directions (forward or backward) and the two orthogonal polarizations of a light beam. We demonstrate that one-way transparency can be realized for spin-wave excitations with sufficiently strong optical magnetoelectric effect. Furthermore, the transparent and absorbing directions of light propagation can be reversed by external magnetic fields. This magnetically controlled optical-diode function of magnetoelectric multiferroics may open a new horizon in photonics. Nature offers a plethora of dichroic materials whose colour is different for two specific polarizations of the transmitted light. Dichroism generally appears in media that are not isotropic and provides information about their symmetry. Linear dichroism (absorption difference for two orthogonal linear polarizations of a light beam) emerges in materials where the symmetry is lower than cubic, while circular dichroism (absorption difference for the two circular polarizations) is observed in materials with finite magnetization or chiral structure. In all these cases, the four transverse wave solutions of the Maxwell equations for a given axis of light propagation group into two pairs, where each pair contains two counter-propagating waves (± k ) with the same absorption coefficient [1] , [2] . In materials with simultaneously broken spatial inversion and time reversal symmetry this two-fold ± k directional degeneracy of the Maxwell equations can be lifted and each of the four waves may be absorbed with a different strength [3] , [4] , [5] , [6] , [7] . We call this phenomenon quadrochroism and the corresponding materials quadrochroic or four-coloured media . Following the early prediction of ± k directional anisotropy [4] , [8] , [9] and experimental observation [10] , [11] of weak directional anisotropy effects, recent studies on multiferroics found strong directional dichroism (difference in the absorption coefficient for counter-propagating light beams) in the GHz-THz [6] , [12] , [13] , [14] , [15] and visible spectral range [16] , [17] , [18] as a hallmark of quadrochroism. Magnetoeletric multiferroic materials simultaneously exhibit two ferroic properties in a single phase, namely they are both ferromagnetic and ferroelectric [19] . In a broader sense, ferroelectrics concurrently hosting ferrimagnetic or antiferromagnetic order are also referred to as magnetoelectric multiferroics. When the coexisting magnetic and electric order parameters are intimately coupled to produce the static magnetoelectric effect, electric polarization can be generated by a magnetic field and magnetization appears in response to an electric field [20] , [21] . In magnetoelectric multiferroics, the coupling between the electric and magnetic states also leads to the dynamical or optical magnetoelectric effect described by the response functions ( ω ) and ( ω ) [4] , [5] , [6] , [12] , [13] , [22] . Consequently, oscillating magnetization and polarization ( M ω and P ω ) are induced by the electric and magnetic components of light ( E ω and H ω ), respectively, besides the conventional terms arising from the dielectric permittivity ( ) and magnetic permeability ( ) tensors: M ω =[ ( ω )−1] H ω + ( ω ) E ω and P ω = 0 [ ( ω )−1] E ω + ( ω ) H ω . The static magnetoelectric effect has been widely proposed to form the basis for a fundamentally new type of memory devices by realizing a fast low-power electrical write operation and a non-destructive non-volatile magnetic read operation [23] , [24] , [25] . Here we show that its dynamical analogue, the optical magnetoelectric effect, may generate quadrochroism and give rise to new optical functionalities such as magnetically controllable one-way transparency. We argue that quadrochroism is an inherent property of magnetoelectric multiferroics. Quadrochroism induced by the optical magnetoelectric effect Optical properties of magnetoelectric media can be described phenomenologically by solving the Maxwell equations with the generalized constitutive relations quoted above [4] , which yields the following form of the refractive index for a given polarization [12] , [26] : The±signs correspond to wavevectors ± k , while i and j specify the directions of the electric field ( E ω ∥ e i ) and the magnetic field ( H ω ∥ h j ) of light, respectively. The unit vectors e i and h j together with k form a right-handed system. Using i , j subscripts, polarization dependence is also indicated for the refractive index and other scalar quantities such as the absorption and reflectivity coefficients. The second term in Equation 1 shows the key role of the optical magnetoelectric effect in generating quadrochroism by lifting the ± k degeneracy of the Maxwell equations. The derivation of Equation 1 for magnetoelectric materials of various symmetries is given in the Methods section. The optical magnetoelectric effect is exclusively generated by such transitions where both the electric- and magnetic-dipole moments induced by an absorbed photon with energy ħω are finite: that is, the magnetic ( m j ) and electric ( p i ) dipole operators must simultaneously have non-vanishing matrix elements between the ground state |0 and the excited states | n separated by ħω n 0 energy. V is the volume of the system, δ n is the inverse lifetime of the excited state | n , 0 and μ 0 are respectively the permittivity and the permeability of the vacuum. ( ω ) and ( ω ) are the sum of terms with the real ( ℜ ) and the imaginary ( ℑ ) parts of the matrix element products, respectively, and do not correspond to the real and imaginary parts of the total ( ω ). This classification is based on the time parity of the two parts, ( ω ) changes sign under time reversal and ( ω ) remains invariant, which plays an important role in the peculiar optical phenomena studied here. The time-odd (ω) is solely responsible for the ± k directional anisotropy, i.e., , as the two cross effects are related by the Kubo formula according to and . The static magnetoelectric effect is also governed by , since vanishes in the zero-frequency limit. Equation 2 provides a direct link between the static magnetoelectric effect and the directional anisotropy by pointing to the common microscopic origin of the two phenomena. When the optical magnetoelectric effect is sufficiently strong, a four-coloured material can become fully transparent for a given propagation direction, while it still absorbs light travelling in the opposite direction as depicted in Fig. 1a . Specific to an excitation with a given resonance energy ħω n 0 and polarization ( e i , h j ), we define the magnetoelectric ratio as . 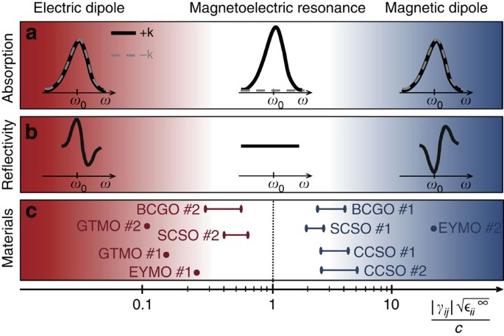Figure 1: One-way transparency at magnetoelectric resonances. Optical properties characteristic to pure electric-dipole, mixed magnetoelectric and pure magnetic-dipole excitations corresponding to different values of the magnetoelectric ratio, γi,j. (a) Counter-propagating beams are absorbed with the same strength in case of pure electric (red region) and magnetic (blue region) dipole transitions as illustrated by the two absorption peaks at ω0labelled with +k(black line) and −k(grey dashed line). When approaching the limit of ideal magnetoelectric resonance (white region), where |γi,j|=c/, the material tends to show one-way transparency. (b) Electric- and magnetic-dipole transitions emerge with opposite line shapes in the normal-incidence reflectivity spectrum, while an ideal magnetoelectric resonance remains hidden. (c) Magnetoelectric ratio for magnon modes with strong ±kdirectional anisotropy observed in multiferroic Ca2CoSi2O7(CCSO), Sr2CoSi2O7(SCSO), Ba2CoGe2O7(BCGO), Gd0.5Tb0.5MnO3(GTMO)15and Eu0.55Y0.45MnO3(EYMO)14. For the first three compounds studied here, the intervals over which the magnetoelectric ratio changes with application of magnetic fields (B=0–12 T) are indicated by bars. For the other two compounds only approximate values are shown based on previous studies. The assignment of the modes is specified in the main text andFig. 3. The γi,jvalues and their field dependence for the different modes are given in theSupplementary Fig. 1. For a magnetoelectric resonance separated from other excitations, the absorption, given by the imaginary part of the refractive index, vanishes for either forward or backward propagation, that is, the resonance shows one-way transparency if Figure 1: One-way transparency at magnetoelectric resonances. Optical properties characteristic to pure electric-dipole, mixed magnetoelectric and pure magnetic-dipole excitations corresponding to different values of the magnetoelectric ratio, γ i , j . ( a ) Counter-propagating beams are absorbed with the same strength in case of pure electric (red region) and magnetic (blue region) dipole transitions as illustrated by the two absorption peaks at ω 0 labelled with + k (black line) and − k (grey dashed line). When approaching the limit of ideal magnetoelectric resonance (white region), where | γ i , j |= c / , the material tends to show one-way transparency. ( b ) Electric- and magnetic-dipole transitions emerge with opposite line shapes in the normal-incidence reflectivity spectrum, while an ideal magnetoelectric resonance remains hidden. ( c ) Magnetoelectric ratio for magnon modes with strong ± k directional anisotropy observed in multiferroic Ca 2 CoSi 2 O 7 (CCSO), Sr 2 CoSi 2 O 7 (SCSO), Ba 2 CoGe 2 O 7 (BCGO), Gd 0.5 Tb 0.5 MnO 3 (GTMO) [15] and Eu 0.55 Y 0.45 MnO 3 (EYMO) [14] . For the first three compounds studied here, the intervals over which the magnetoelectric ratio changes with application of magnetic fields ( B =0–12 T) are indicated by bars. For the other two compounds only approximate values are shown based on previous studies. The assignment of the modes is specified in the main text and Fig. 3 . The γ i , j values and their field dependence for the different modes are given in the Supplementary Fig. 1 . Full size image where c is the speed of light in vacuum, is the dielectric permittivity for the given light polarization due to optical transitions at higher frequencies. Note that one-way transparency is only possible when the interference between the magnetic- and electric-dipole matrix elements is perfectly constructive or destructive, that is, γ i , j is purely real. Correspondingly, the ± signs refer to the two cases when the polarization and the magnetization simultaneously induced by the electromagnetic field oscillate with zero and π phase difference, respectively. Note that in CGS units Equation 3 has the form γ i , j =± , hence, the magnetic- and electric-dipole matrix elements must be of the same order of magnitude to approach the one-way transparency. (For technical details see the Methods section.) Although directional anisotropy is not manifested in the normal-incidence reflectivity of a vacuum-material interface, the one-way transparency of a bulk material can still be accompanied by a peculiar behaviour of the normal-incidence reflectivity, namely the magnetoelectric resonance remains hidden in the reflectivity spectrum, R (ω). Purely electric- and magnetic-dipole transitions appear in the reflectivity spectrum with opposite line shapes according to the Fresnel formula R i , j = as schematically shown in Fig. 1b . Thus, the relative strength of magnetic and electric susceptibilities for a given transition determines the shape of R ( ω ) near the resonance. When the condition |γ i , j |= c / is fulfilled, the reflectivity spectrum is featureless at the resonance with the constant value of R i , j = as if there were no resonance present in that frequency range. Multiferroic character of Ca 2 CoSi 2 O 7 This compound has a non-centrosymmetric tetragonal structure [27] , [28] where Co 2+ cations with S =3/2 spin form square-lattice layers stacked along the tetragonal [001] axis. The static magnetic and magnetoelectric properties of Ca 2 CoSi 2 O 7 (refs 29 , 30 ), as shown in Fig. 2 , resemble the properties of Ba 2 CoGe 2 O 7 (refs 31 , 32 , 33 , 34 , 35 ) and Sr 2 CoSi 2 O 7 (ref. 36 ). This material undergoes an antiferromagnetic ordering below T N =5.7 K with a small ferromagnetic moment ( M ). In the ordered state, the spins likely form a coplanar structure within the tetragonal planes similarly to the case of Ba 2 CoGe 2 O 7 (refs 37 , 38 ). Below T N , magnetic field applied along the [110] (or ) axis in the tetragonal plane induces ferroelectric polarization ( P ) along the [001] direction, which changes sign at B ≈12 T accompanied by an anomaly in the magnetization. The rotation of B =5 T magnetic field within the tetragonal plane results in a nearly sinusoidal modulation of P with zero crossings for field pointing along the [100] and [010] axes. The variation of M is less than 5% implying that in-plane magnetic anisotropies, due to for example, small orthorhombicity of the crystal structure, become negligible in this field range. On this basis, we expect that the magnetic symmetry of Ca 2 CoSi 2 O 7 can be approximated by the mm ′2′ ( m ′ m 2′) polar point group for B ∥ [110] ( B ∥ ) and by the 22′2′ (2′22′) chiral point group for B ∥ [100] ( B ∥ [010]) similarly to Ba 2 CoGe 2 O 7 (refs 12 , 13 , 35 , 39 ) and Sr 2 CoSi 2 O 7 (ref. 36 ). 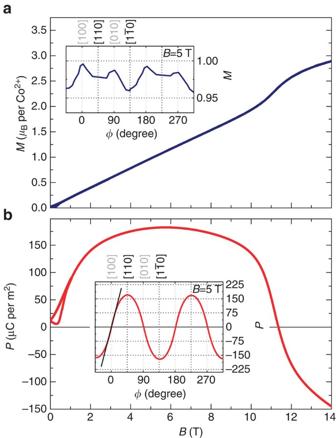Figure 2: Magnetoelectric properties of multiferroic Ca2CoSi2O7atT=2 K. Field dependence of (a) the magnetization (M) and (b) the ferroelectric polarization induced along the tetragonal [001] axis (P) for magnetic fields parallel to the [110] direction. There is a hysteresis in both quantities for fields <1T. The insets display the angular dependence of the magnetization and polarization when a magnetic field ofB=5 T is rotated within the tetragonal plane. The slope of the black line in the inset of panelbis proportional to the static differential magnetoelectric susceptibility inB=5 T applied parallel to the [100] axis. This slope changes sign atB≈12 T together with the sign reversal of the static polarization. Figure 2: Magnetoelectric properties of multiferroic Ca 2 CoSi 2 O 7 at T =2 K. Field dependence of ( a ) the magnetization (M) and ( b ) the ferroelectric polarization induced along the tetragonal [001] axis ( P ) for magnetic fields parallel to the [110] direction. There is a hysteresis in both quantities for fields <1T. The insets display the angular dependence of the magnetization and polarization when a magnetic field of B =5 T is rotated within the tetragonal plane. The slope of the black line in the inset of panel b is proportional to the static differential magnetoelectric susceptibility in B =5 T applied parallel to the [100] axis. This slope changes sign at B ≈12 T together with the sign reversal of the static polarization. Full size image Quadrochroism in Ca 2 CoSi 2 O 7 , Sr 2 CoSi 2 O 7 and Ba 2 CoGe 2 O 7 Former studies on Ba 2 CoGe 2 O 7 have demonstrated the role of magnetoelectric phenomena in the THz optical properties of this material and reported about strong directional dichroism of magnon modes [12] , [13] , [22] , [40] , [41] . Here, we investigate the four-coloured nature of magnons and the possibility to observe one-way transparency in the THz frequency range (0.2−2 THz) on single crystals of Ca 2 CoSi 2 O 7 , Sr 2 CoSi 2 O 7 and Ba 2 CoGe 2 O 7 . Since the ( ω ) magnetoelectric tensor component responsible for the directional anisotropy has odd time parity, reversing the direction of an applied static magnetic field is equivalent to the reversal of light propagation direction. Therefore, we fixed the propagation direction and recorded the absorption spectra ( α ) in magnetic fields parallel and antiparallel to the propagation direction (± B ) for two orthogonal polarizations as shown in Fig. 3 . 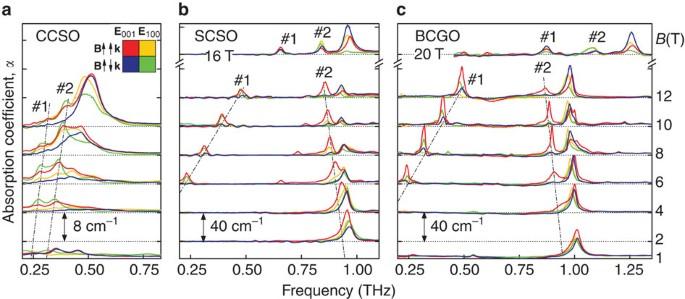Figure 3: Quadrochroic magnons in multiferroics. THz absorption spectra of (a) Ca2CoSi2O7(CCSO), (b) Sr2CoSi2O7(SCSO) and (c) Ba2CoGe2O7(BCGO) measured in magnetic fieldsB∥k∥[010] atT=4 K. The spectra are shifted proportional to the magnitude of the field, which is indicated by the right vertical axis common for each panel. The distance between horizontal grid lines is indicated in each panel. Spectra recorded in the four cases, that is, for beams propagating along and opposite to the magnetic field direction in two orthogonal polarizationsEω∥[001] andEω∥[100], are plotted with four different colours as explained in the inset of panela. For each compound, magnon modes with the strongest ±kdirectional dichroism are indicated with dash-dotted lines and labelled as #1 and #2.Figure 1and the main text refer to these modes in polarizationEω∥[001]. Note that directional dichroism changes sign for some of the modes aroundB≈16 T in SCSO and within the range ofB=12–20 T in BCGO. Similar tendency can be followed inFig. 4for CCSO. Figure 3: Quadrochroic magnons in multiferroics. THz absorption spectra of ( a ) Ca 2 CoSi 2 O 7 (CCSO), ( b ) Sr 2 CoSi 2 O 7 (SCSO) and ( c ) Ba 2 CoGe 2 O 7 (BCGO) measured in magnetic fields B ∥ k ∥ [010] at T =4 K. The spectra are shifted proportional to the magnitude of the field, which is indicated by the right vertical axis common for each panel. The distance between horizontal grid lines is indicated in each panel. Spectra recorded in the four cases, that is, for beams propagating along and opposite to the magnetic field direction in two orthogonal polarizations E ω ∥ [001] and E ω ∥ [100], are plotted with four different colours as explained in the inset of panel a . For each compound, magnon modes with the strongest ± k directional dichroism are indicated with dash-dotted lines and labelled as #1 and #2. Figure 1 and the main text refer to these modes in polarization E ω ∥ [001]. Note that directional dichroism changes sign for some of the modes around B ≈16 T in SCSO and within the range of B =12–20 T in BCGO. Similar tendency can be followed in Fig. 4 for CCSO. Full size image While the static magnetic and magnetoelectric properties of these three compounds show close similarities, magnon modes in Ca 2 CoSi 2 O 7 differ from the magnons observed for the other two compounds in their location, strength and field dependence. Irrespective of these differences, most of the magnon modes show strong quadrochroic character in each compound, that is, the strength of light absorption is different for all the four cases: the two polarizations and the two (± k ) propagation directions. For certain modes one-way transparency is closely realized as the absorption coefficient is nearly zero for light propagating along a given direction, while the absorption remains strong for counter-propagating light beams with the same polarization. Furthermore, in each compound the sign of directional dichroism is reversed for some of the resonances within the field range of B =12–20 T. Next, we show that the directional dichroism observed in Fig. 3 is the consequence of the magnetically induced chirality as previously proposed for Ba 2 CoGe 2 O 7 , where magnetic switching between the two chiral enantiomers (22′2′ and 2′22′) has been verified by the detection of natural circular dichroism for the magnon modes [13] . For this purpose, we studied the effect of the magnetic field orientation on the absorption spectra of Ca 2 CoSi 2 O 7 . The sign of the directional dichroism is reversed by changing the orientation of the sample from B ∥ [100] to B ∥ [010] via π/2 rotation of the crystal around the tetragonal axis (compare spectra in Fig. 4a,b ). On the other hand, rotating the crystal by π around any of the [100], [010] and [001] axes during the measurement leaves the absorption spectra unchanged. These observations support our assignment that the symmetry of these materials corresponds to the 22′2′ and 2′22′ chiral point group for B ∥ [100] and B ∥ [010], respectively. Thus, the directional dichroism observed here in Faraday configuration ( B ∥ k ) is the manifestation of chirality. 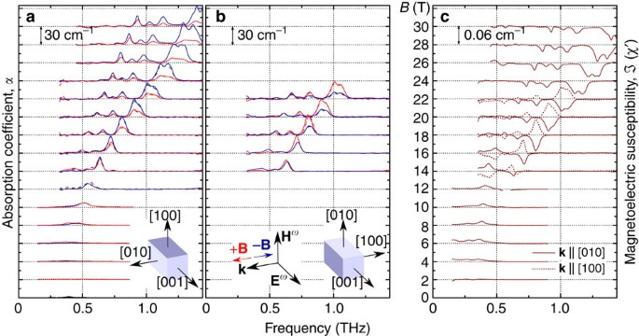Figure 4: Directional dichroism of magnon modes and magnetic switching of chirality in Ca2CoSi2O7. (a,b) Absorption spectra measured in Faraday configuration, that is, forB∥k, in magnetic fieldsB=0–30 T atT=2 K. The spectra are shifted vertically proportional to the magnitude of the field and the distance between horizontal grid lines is indicated in each panel. The relative orientation of the static magnetic field, the polarization and the propagation direction of light, common for all spectra in the figure, are shown in panelb, while the corresponding sample orientations are specified in each panel. In panelathe polarization configuration isEω∥[001],Hω∥[100] andk∥[010], while in panelbthe sample is rotated by π/2 around the [001] axis. Red and blue spectra correspond to light propagation along and opposite to the magnetic field, respectively. The modes exhibit strong directional dichroism. Measurements shown in panelsaandbwere repeated afterπrotations of the sample around the [100], [010] and [001] axes. The corresponding spectra plotted with dashed lines nearly coincide with the original ones in the whole frequency range. The imaginary part of the optical magnetoelectric susceptibility (ℑ{χ′}), which is proportional to the directional dichroism, is plotted in panelc.ℑ{χ′} changes sign between the two configurations shown in panelsaandbdue to the magnetic switching between the left- and right-handed form of the material. Figure 4: Directional dichroism of magnon modes and magnetic switching of chirality in Ca 2 CoSi 2 O 7 . ( a , b ) Absorption spectra measured in Faraday configuration, that is, for B ∥ k , in magnetic fields B =0–30 T at T =2 K. The spectra are shifted vertically proportional to the magnitude of the field and the distance between horizontal grid lines is indicated in each panel. The relative orientation of the static magnetic field, the polarization and the propagation direction of light, common for all spectra in the figure, are shown in panel b , while the corresponding sample orientations are specified in each panel. In panel a the polarization configuration is E ω ∥ [001], H ω ∥ [100] and k ∥ [010], while in panel b the sample is rotated by π/2 around the [001] axis. Red and blue spectra correspond to light propagation along and opposite to the magnetic field, respectively. The modes exhibit strong directional dichroism. Measurements shown in panels a and b were repeated after π rotations of the sample around the [100], [010] and [001] axes. The corresponding spectra plotted with dashed lines nearly coincide with the original ones in the whole frequency range. The imaginary part of the optical magnetoelectric susceptibility ( ℑ {χ′}), which is proportional to the directional dichroism, is plotted in panel c . ℑ { χ ′} changes sign between the two configurations shown in panels a and b due to the magnetic switching between the left- and right-handed form of the material. Full size image As a more fundamental quantity, the optical magnetoelectric susceptibility spectra calculated from the absorption spectra of counter-propagating beams with a given polarization according to ℑ { ( ω )}≈ are plotted in Fig. 4c . ℑ { } has opposite signs in the left- and right-handed forms of the material, which are established by magnetic fields pointing parallel to the [100] and [010] crystallographic axes, respectively. A summary of the ℑ { ( ω )} spectra obtained for the three materials is given in Fig. 5 . In all the three cases, the static magnetic field was applied parallel to the [100] axis, and two independent components of the magnetoelectric tensor have been evaluated from the absorption spectra measured with the two orthogonal polarizations of light. 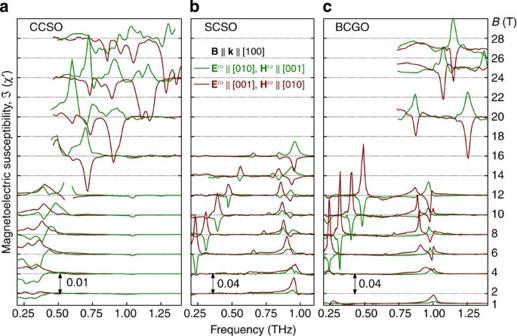Figure 5: Magnetic field dependence of the optical magnetoelectric susceptibility. ℑ{χ′(ω)} spectra of (a) Ca2CoSi2O7(CCSO), (b) Sr2CoSi2O7(SCSO) and (c) Ba2CoGe2O7(BCGO). Indices of χ′(ω) are omitted in the figure. Instead, the two polarization configurations are specified by colours in the figure. Following the notation introduced in Equation 1, brown and green spectra correspond to the components χ′[010],[001]and χ′[001],[010]as they are obtained from absorption spectra measured in polarizations (Eω∥[001],Hω∥[010]) and (Eω∥[010],Hω∥[001]), respectively. Figure 5: Magnetic field dependence of the optical magnetoelectric susceptibility. ℑ {χ′( ω )} spectra of ( a ) Ca 2 CoSi 2 O 7 (CCSO), ( b ) Sr 2 CoSi 2 O 7 (SCSO) and ( c ) Ba 2 CoGe 2 O 7 (BCGO). Indices of χ′( ω ) are omitted in the figure. Instead, the two polarization configurations are specified by colours in the figure. Following the notation introduced in Equation 1, brown and green spectra correspond to the components χ′ [010],[001] and χ′ [001],[010] as they are obtained from absorption spectra measured in polarizations ( E ω ∥ [001], H ω ∥ [010]) and ( E ω ∥ [010], H ω ∥ [001]), respectively. Full size image When the crystal is rotated by π/4 around the [001] axis, that is, the direction of the external magnetic field is changed from B ∥ [100] to B ∥ [110], the material is expected to become not chiral but polar. This was experimentally verified by the lack of ± k directional anisotropy in Faraday configuration as shown for Ca 2 CoSi 2 O 7 and Sr 2 CoSi 2 O 7 in the Supplementary Fig. 2 . In this case, the spin excitations show no directional dichroism because the magnetoelectric ratio, γ i , j , is either zero or infinity for each resonance when ( E ω ∥ [001], H ω ∥ ) and ( E ω ∥ , H ω ∥ [001]). Hence, the modes loose their quadrochroic character and become ordinary dichroic transitions. One-way transparency of magnetoelectric excitations As clear from Equation 3, one-way transparency in a finite spectral range is not prohibited by any fundamental law of nature. While the conventional magnon modes are only magnetic-dipole active, the spin-wave excitations in multiferroics can have a magnetoelectric (both electric- and magnetic-dipole) character [6] , [12] , [13] , [14] , [15] , [22] , [26] and be even dominantly electric-dipole active [42] , [43] , [44] , [45] , [46] , [47] , [48] , [49] . Since the ratio of the matrix elements can be controlled via the spin system and is mainly determined by the lattice vibrations, one-way transparency can be achieved by synthesis of tailored material. The magnetoelectric ratio for a separate transition can be calculated from the absorption measured for counter-propagating beams with a given polarization, and : Here, the upper/lower sign corresponds to the case when the transition is located at the magnetic/electric-dipole side of the border of one-way transparency, which can be determined from polarized reflectivity spectra as explained earlier or by the systematic polarization dependence of the absorption spectra. (See Methods section for the derivation of Equation 4.) Figure 1 shows the magnetoelectric ratio, γ i , j , for magnon modes with strong directional anisotropy in Ca 2 CoSi 2 O 7 , Sr 2 CoSi 2 O 7 , Ba 2 CoGe 2 O 7 and in two other multiferroics Gd 0.5 Tb 0.5 MnO 3 (ref. 15 ) and Eu 0.55 Y 0.45 MnO 3 (ref. 14 ). Note that the absorption coefficient for counter-propagating light beams differs by more than one order of magnitude for modes located in the region of 0.5<|γ i , j |<2. The selected modes are separated from other transitions, hence, their magnetoelectric ratio can be determined according to Equations 3 and 4. For Ca 2 CoSi 2 O 7 , Sr 2 CoSi 2 O 7 and Ba 2 CoGe 2 O 7 the labelling of the modes follows the notation used in Fig. 3 . GTMO #1 and EYMO #1 are the lowest-energy spin-current driven electromagnon modes in Gd 0.5 Tb 0.5 MnO 3 (ref. 15 ) and Eu 0.55 Y 0.45 MnO 3 (ref. 14 ), respectively. GTMO #2 is the exchange-striction induced electromagnon [42] , [44] , [46] and EYMO #2 is the conventional antiferromagnetic resonance [50] , both located at ≈0.6–0.7 THz (the selection rules for these transitions are as specified in refs 14 , 15 ). The magnetoelectric ratio can be unambiguously determined from the directional anisotropy data together with the systematic polarization dependence of the absorption spectra for the modes in Ba 2 CoGe 2 O 7 (refs 12 , 13 , 40 ) and for the higher-energy modes in Gd 0.5 Tb 0.5 MnO 3 (refs 15 , 44 , 46 ) and Eu 0.55 Y 0.45 MnO 3 (refs 14 , 50 ). The dominantly magnetic- and electric-dipole characters of modes BCGO #1 and BCGO #2, respectively, are in agreement with the theoretical predictions [22] , [40] . Because of the close similarity between the magnon spectra of Sr 2 CoSi 2 O 7 and Ba 2 CoGe 2 O 7 , we use the same assignment for Sr 2 CoSi 2 O 7 . The spin excitations in Ca 2 CoSi 2 O 7 are tentatively assigned to the magnetic-dipole side of the γ i , j = c / boundary, while the spin-current driven mode in Gd 0.5 Tb 0.5 MnO 3 and Eu 0.55 Y 0.45 MnO 3 is assumed to be at the electric-dipole side. Note that the selected magnon modes in Sr 2 CoSi 2 O 7 , Ca 2 CoSi 2 O 7 and Ba 2 CoGe 2 O 7 show nearly one-way transparency as also evident from Fig. 3 . DC magnetoelectric effect governed by directional dichroism As already discussed in the context of Equation 2, directional optical anisotropy and static magnetoelectric effect share a common microscopic origin. Their relation can be quantitatively formulated by the Kramers-Kronig transformation when taking the zero-frequency limit: Hence, the static magnetoelectric coefficient is proportional to the integral of the directional dichroism over the whole frequency range. Due to the ω′ 2 denominator, the main contributions to the integral come from the lowest-frequency magnetoelectric excitations, for example, from magnon modes. We note that the second equality in Equation 5 holds only if ( ω )≡0, that is, 0| m j | n n | p i |0 is real. This is indeed the case for multiferroic compounds belonging to many magnetic point groups such as 42′2′, 22′2′, 2′, mm ′2′, mmm ′. The connection between the static and optical magnetoelectric phenomena is also manifested in the present materials. The magnetically induced ferroelectric polarization together with the differential magnetoelectric effect (indicated for Ca 2 CoSi 2 O 7 in the caption of Fig. 2b ) change sign at B ≈12 T, 16 T and 15 T in Ca 2 CoSi 2 O 7 , Sr 2 CoSi 2 O 7 and Ba 2 CoGe 2 O 7 , respectively [31] , [36] . Since directional dichroism is governed by the same differential magnetoelectric effect in the optical region, the sign of the integral in Equation 5 should simultaneously be reversed. Accordingly, in the same magnetic field region, we observed the sign reversal of the directional dichroism for most of the modes in each compound. The optical magnetoelectric effect measures the interference between the electric polarization and the magnetization that are simultaneously induced in the light absorption processes. The interference term, that is, 0| m j | n n | p i |0 matrix element product, is sensitive to the relative orientation of the static electric polarization and the static magnetization in multiferroics. Indeed directional dichroism can emerge in multiferroics where the ferroelectric polarization is not parallel to the magnetization [7] , [12] , [14] , [15] , in magnets with ferrotoroidic order [7] , and in the present case of magnetically induced chirality. Therefore, the measurement of directional anisotropy may be applied for spatial mapping of multiferroic domain structures, a capability that has been considered to be the privilege of non-linear optical techniques such as the optical second harmonic generation [51] , [52] , [53] , [54] . As a more fundamental issue, the optical magnetoelectric susceptibility determined from the directional dichroism spectrum can help to distinguish between possible microscopic mechanisms of magnetoelectric coupling in multiferroics. The directional dichroism observed for magnon modes in Ba 2 CoGe 2 O 7 has been closely reproduced by the spin-dependent metal-ligand hybridization model [13] previously proposed to describe the static magnetoelectric properties of this compound. In the spin-cycloidal state of perovskite manganites, directional dichroism is strong for the low-energy mode induced by the spin-current mechanism (GTMO #1 and EYMO #1 in Fig. 1 ), while it is weak for the higher-energy mode driven by magnetostriction (GTMO #2) [14] , [15] . This is in agreement with the expected magnetoelectric nature of GTMO #1 and EYMO #1 magnon modes and the dominantly electric-dipole character of GTMO #2 magnon mode [6] , [14] , [15] , [42] , [43] , [45] . We have demonstrated that quadrochroism generated by the optical magnetoelectric effect in multiferroics is an inherent property of the spin-wave excitations located in the THz spectral range. Depending on the ratio of light-induced oscillating magnetization and electric polarization, these excitations can exhibit one-way transparency in specific light polarization. As another consequence of quadrochroism, directional dichroism is not cancelled but remains finite for unpolarized light. Moreover, an excitation showing one-way transparency remains hidden in the reflectivity. Recently, directional anisotropy has been predicted [55] and also observed [56] for the spin excitations of skyrmion crystals at GHz frequencies. Besides spin excitations in the GHz-THz spectral range, the optical magnetoelectric effect can strongly influence the optical properties of multiferroics in the infrared-visible region. Crystal field transitions of the d or f shell electrons of magnetic ions show strong directional anisotropy as was observed in multiferroic CuB 2 O 4 (refs 16 , 17 ) and (Cu,Ni)B 2 O 4 (ref. 18 ). Although the crystal-field excitations predominantly have an electric-dipole character, strong spin-orbit interaction can tune their magnetoelectric ratio closer to γ i , j = c / . In contrast to the common belief that lattice vibrations are purely electric-dipole active transitions, the optical magnetoelectric effect can also emerge for phonon modes in multiferroics as has been reported recently for the magnetoelectric atomic rotations in Ba 3 NbFe 3 Si 2 O 14 (ref. 57 ). To complete the list of excitations, we recall that directional dichroism was first observed for excitonic transitions of the polar semiconductor CdS in external magnetic fields by Hopfield and Thomas [58] in 1960. Since the whole zoo of spin, orbital and lattice excitations can exhibit optical magnetoelectric effect in multiferroics, directional control of light in these materials may work over a broad spectrum of the electromagnetic radiation from the THz range to the visible region. On the other hand, the presence of static magnetization and electric polarization in multiferroics facilitates the switching between the transparent and absorbing directions of light propagation via static magnetic or electric fields. The one-way transparency observed here emerges for ‘conventional’ (zone-center) magnon modes of multiferroic compounds with simple antiferromagnetic order, hence, such optical-diode function is expected to be present in a broad variety of multiferroics. Polarized THz absorption spectroscopy For the study of polarized absorption in magnetic fields up to 30 T, we used Fourier transform spectroscopy. The measurement system for the B =0–12 T region is based on a Martin-Puplett interferometer, a mercury arc lamp as a light source and a Si bolometer cooled down to 300 mK as a light intensity detector. This setup covers the spectral range 0.13–6 THz with a maximum resolution of 0.004 THz. The polarization of the beam incident to the sample is set by a wire-grid polarizer, while the detection side (light path from the sample till the detector) is insensitive to the polarization of light. Experiments up to 30 T were carried out in the High Field Magnet Laboratory in Nijmegen, where a Michaelson interferometer is used together with a 1.6 K Si bolometer providing a spectral coverage of 0.3–6 THz. All the measurements were carried out in Faraday configuration, that is, by applying magnetic fields (anti)parallel to the direction of light propagation using oriented single crystal pieces with the typical thickness of 1 mm. The crystals were grown by a floating-zone method and were characterized by magnetization and ferroelectric polarization experiments before the optical study [31] . Formulae for quadrochroism The quadrochroism of spin excitations located in the long-wavelength region of light can be described by the Maxwell’s equations by introducing the dynamical magnetoelectric effects into the constitutive relations: The microscopic form of the dielectric permittivity ( ) and magnetic permeability ( ) is given by the Kubo formula: Here, and are the sum of terms with the real ( ℜ ) parts of the matrix element products (also including δ ji and δ ji , respectively) while, and are the sum of terms with the imaginary ( ℑ ) parts of the matrix element products. In contrast to the parity of the magnetoelectric tensor introduced in Equation 2, ( ) is invariant and ( ) changes sign under time reversal. is the background dielectric constant from modes located at higher frequencies than the studied frequency window, while magnetic permeability contribution from higher-frequency excitations is neglected being usually much smaller than unity. Among crystals exhibiting ± k directional anisotropy, the highest symmetry ones are the chiral materials with the 432 cubic point group when magnetization develops along one of their principal axes. In this case, their magnetic point symmetry is reduced to 42′2′ where ′ means the time-reversal operation. The fourfold rotational symmetry is preserved around the direction of the magnetization chosen as the y -axis in the following. According to Neumann’s principle, for materials belonging to the point group the dynamical response tensors have the following form: and the general relation yields in the present symmetry . By solving the Maxwell equations for propagation parallel and antiparallel to the magnetization direction (± k ∥ y ), one obtains the following refractive indices for the left (l) and right (r) circularly polarized eigenmodes: The reflectivity of an interface between the vacuum and a material with 42′2′ symmetry can be determined from the Maxwell equations in the usual way by using the boundary conditions. For normal incidence the components of the magnetoelectric tensor do not appear in the reflectivity and one can reproduce the general expression: where Z l / r = Z 0 and Z 0 are the surface impedance of the interface and the impedance of vacuum, respectively. Keeping only the leading term in the surface impedance, that is, Z = Z 0 for polarization E ω ∥ e i and H ω ∥ h j , the expression for the normal-incidence reflectivity given above is generally valid for materials belonging to other magnetic point groups as well. When the symmetry is reduced to , as is the case in the magnetically induced chiral state of Ca 2 CoSi 2 O 7 and Ba 2 CoGe 2 O 7 , the equivalence of x - and z -axis does not hold anymore. Consequently the form of the tensors changes and the eigenmodes become elliptically polarized. Since the (100) plane studied for these materials shows strong linear dichroism/birefringence because of their crystal structure (with the dielectric constant ∞ ≈12 and 8 for polarizations along the optical axes [100] and [001], respectively, as determined from transmission data), the eigenmodes are expected to be nearly linearly polarized. The approximate form of the refractive index, when keeping only the time-reversal odd components of and the time-reversal even components in and (that is, neglecting polarization rotation): In a broad class of orthorhombic multiferroics, the magnetization and ferroelectric polarization are perpendicular to each other. Choosing the magnetization and polarization parallel to the y -axis and z -axis, respectively, the magnetic point group is the . In this case, the form of and tensors is the same as in but the magnetoelectric tensors become different: For propagation perpendicular both to the direction of the magnetization and the ferroelectric polarization (± k ∥ x ), the refractive indices for the two linearly polarized eigenmodes are: While in the lowest-order approximation the general formulae are and as given in Equation 1, quadrochroism can be generated by other higher-order terms, such as , that are odd both in time reversal and spatial inversion. Note that ′ and ′′ correspond to the part of being odd and even under time reversal, respectively, while the situation is reversed for and . The criterion for one-way transparency We calculate the absorption coefficient in the vicinity of a separate magnetoelectric resonance, that is, when the photon with the frequency ω = ω n 0 resonantly excites the |0 → | n transition. When using the Kubo formula for , and , the refractive index for a given polarization, , has the following form: where the square root in the first term is expanded up to the second order. Then, the absorption coefficient vanishes for one direction, that is, either =0 or =0, if where c is the speed of light in vacuum, is the dielectric permittivity for the given polarization due to other optical transitions and ξ= ℜ {γ i,j }/|γ i,j |. Note that one-way transparency is only possible when γ i , j is purely real corresponding to ξ =+ 1 or −1 and the formula simplifies to |γ i , j |= c / as given in Equation 3. Note that γ i , j is real when =0, which is the case for many multiferroic materials belonging to different magnetic point groups including 42′2′ (Nd 5 Si 4 ) (ref. 59 ), 22′2′ (CuB 2 O 4 ) (ref. 16 ), 2′ (LiCoPO 4 ) (ref. 60 ), mm ′2′ (GaFeO 3 ) (ref. 61 ), mmm ′ (LiNiPO 4 ) (ref. 62 ). When γ ij is real, Equation 4 can be straightforwardly derived from Equation 21. When the condition of one-way transparency holds for a separate resonance in a given polarization , the surface impedance does not change near the resonance and has the frequency independent Z =1/ value. Thus, the reflectivity also coincides with the background value R = . How to cite this article: Kézsmárki, I. et al. One-way transparency of four-coloured spin-wave excitations in multiferroic materials. Nat. Commun. 5:3203 doi: 10.1038/ncomms4203 (2014).